Cloning southern corn rust resistant geneRppKand its cognate geneAvrRppKfromPuccinia polysora Broad-spectrum resistance has great values for crop breeding. However, its mechanisms are largely unknown. Here, we report the cloning of a maize NLR gene, RppK , for resistance against southern corn rust (SCR) and its cognate Avr gene, AvrRppK , from Puccinia polysora (the causal pathogen of SCR). The AvrRppK gene has no sequence variation in all examined isolates. It has high expression level during infection and can suppress pattern-triggered immunity (PTI). Further, the introgression of RppK into maize inbred lines and hybrids enhances resistance against multiple isolates of P. polysora , thereby increasing yield in the presence of SCR. Together, we show that RppK is involved in resistance against multiple P. polysora isolates and it can recognize AvrRppK, which is broadly distributed and conserved in P. polysora isolates. Maize ( Zea mays L) is one of the crops with the highest production and a major source of calories and proteins for livestock and humans worldwide. However, the grain yield and quality of maize are seriously reduced by many diseases around the world. The most efficient way to control these diseases is to develop maize lines carrying resistance genes. The identification and cloning of resistance genes are critical steps toward that goal. However, only sixteen resistance genes ( Hm1 , Htn1 , Ht2 , Ht3 , Rp1-D21 , RppC , RabGD1α , ZmABP1 , ZmAuxRP1 , ZmCCoAOMT2 , ZmCCT , ZmFBL41 , ZmMM1 , ZmREM1.3 , ZmTrxh , ZmWAK ) have been cloned from maize [1] , [2] , [3] , [4] , [5] , [6] , [7] , [8] , [9] , [10] , [11] , [12] , [13] , [14] , [15] , and very few of them have been proven to have breeding value. Plant innate immunity consists of pattern-triggered immunity (PTI) and effector-triggered immunity (ETI) [16] . PTI is triggered by the recognition of microbial components by cell surface-localized pattern-recognition receptors (PRRs), while ETI is activated by the recognition of microbial effector proteins directly or indirectly by intracellular nucleotide-binding leucine-rich repeat receptors (NLRs) [16] . ETI activates more rapid and stronger immunity than PTI [17] , [18] , although they share similar downstream cellular responses [19] , [20] . Therefore, the deployment of NLR genes in crop cultivars has been the major approach for improving disease resistance in crop breeding [21] . Unfortunately, the resistance conferred by NLR genes is often not durable in the field because of changes in pathogen races. Pathogen races without corresponding effector genes (known as avirulence, Avr , genes) accumulate quickly, and pathogen races may evolve through the mutation or deletion of the corresponding Avr gene, resulting in the breakdown of resistance conferred by NLR genes [16] , [21] , [22] . For example, the Ug99 race group of Puccinia graminis f. sp. tritici has successfully broken through the resistance of wheat cultivars conferred by the Sr31 , Sr24 , Sr36 , and SrTmp resistance genes [23] , [24] , [25] , [26] . To achieve broad-spectrum resistance, the pyramiding of multiple NLR genes has been applied in breeding [22] . For example, the pyramiding of yellow rust resistance genes ( Yr5 and Yr15 or Yr64 and Yr15 ) in wheat resulted in broad-spectrum resistance against all tested stripe rust races [27] , [28] . Another way to obtain broad-spectrum resistance is to deploy NLR genes recognizing core effectors, which are widely distributed in most races of a particular pathogen and are required for their virulence in crops [21] . Although much work has been performed to achieve that goal [29] , [30] , no core effector gene- NLR gene pairs have been identified in major pathogens and crops. Therefore, no direct evidence has been presented to prove that this strategy is practicable. Owing to changes in climate and cropping practices, southern corn rust (SCR) caused by Puccinia polysora UnderW. has become a major maize disease in the USA, Canada, Brazil, and China [31] , [32] , [33] , [34] , [35] . Under favorable conditions, SCR can cause yield losses of more than 50%, which seriously threatens maize production and food security [31] , [32] , [35] , [36] , [37] , [38] . Similar to other rust fungi, P. polysora behaves as an obligate biotroph that only extracts nutrients from living cells. Although eleven maize dominant resistance genes ( Rpp1 to Rpp11 ) and eight maize major resistance QTLs ( RppC , RppCML470 , RppD , RppM , RppP25 , RppQ , RppS , and RppS313 ) against P. polysora have been reported, only RppC was cloned [14] , [31] , [33] , [37] , [39] , [40] , [41] , [42] , [43] , [44] . In this work, we clone a maize CC-NB-LRR gene, RppK , involved in resistance against P. polysora by map-based cloning, and its cognate Avr gene, AvrRppK , from P. polysora . AvrRppK is highly conserved in all tested P. polysora isolates and can suppress chitin-induced PTI. Furthermore, the RppK gene has great value for breeding because maize inbred lines or hybrids introgressed with the RppK gene exhibit stronger resistance against P. polysora and higher yields than those without the RppK gene in the presence of P. polysora . Map-based cloning of RppK K22 is a maize inbred line with durable and complete resistance against SCR in China over the last 30 years (Fig. 1a and Supplementary Fig. 1a ). To study the genetic mechanism underlying its resistance against SCR, K22 was crossed with the susceptible inbred line DAN340 to generate a K22 × DAN340 F 6:7 population [45] , [46] , and the disease phenotypes of these plants were evaluated, based on the SCR disease scale (Supplementary Fig. 1b, c ). QTL analysis identified one major QTL , RppK , on the short arm of chromosome 10 that accounted for 68% of the phenotypic variation in resistance against SCR (Fig. 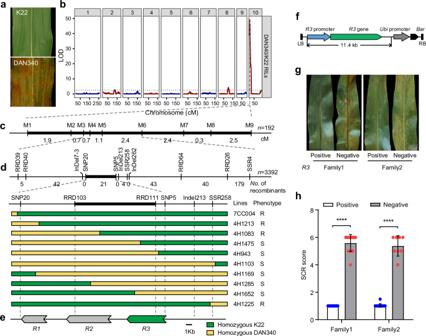Fig. 1: Map-based cloning of theRppKgene, conferring resistance against southern corn rust. aSouthern corn rust (SCR) disease phenotypes of maize inbred lines K22 and DAN340.bSCR-relatedQTLlocations in the genetic population of DAN340/K22 RILs. LOD, logarithm of odds.cThe linkage mapping of theRppKlocus based on 192 families delimited it to the region between markers M3 and M6. The numbers below the black rectangle indicate the relative genetic distance (cM) between markers.dHigh-resolution linkage analysis performed by genotyping 3392 plants of a heterogeneous inbred family (HIF) delimitedRppKto a 15.2 kb interval flanked by markers RRD103 and RRD111. The number of recombinants is shown below the markers. Green segments represent the K22 allele, and yellow segments represent the DAN340 allele. The names of lines and the corresponding phenotypes are provided next to the haplotype. R, resistant; S, susceptible.eTheRppKregion contains three predictedNLRgenes, which encode CC-NB-LRR proteins. Scale bar, 1 kb.fStructure of theR3genomic sequence construct used for generating transgenic maize plants. LB, left border; RB, right border; Bar: Bialaphos Resistance gene. The construct contains the entireR3genomic DNA sequence, including its 3.1 kb promoter region and a 2.4 kb downstream region. The back arrow indicates the Bar gene.g,hThe disease phenotypes and scores of two independent transgenic plant families carrying theR3genomic sequence. Values are means ± SDs;n= 15, 17, 14, and 8 individual plants of positive and negative lines of family 1 and family 2, respectively. ****P< 0.0001 (Student’st-test, two-tailed;P= 1.2596E-15, 5.4354E-07). Source data are provided as a Source Data file. 1b and Supplementary Table 1 ). To fine-map RppK , we genotyped and evaluated the SCR resistance of 402 recombinant lines isolated from 3392 HIF (heterogeneous inbred family)-derived F 2 populations [47] . RppK was mapped to an interval of ~18.3 kb delimited by the markers SNP20 and SNP5 based on the B73 RefGen_v4 genomic sequence (Fig. 1c, d and Supplementary Fig. 2 ). Fig. 1: Map-based cloning of the RppK gene, conferring resistance against southern corn rust. a Southern corn rust (SCR) disease phenotypes of maize inbred lines K22 and DAN340. b SCR-related QTL locations in the genetic population of DAN340/K22 RILs. LOD, logarithm of odds. c The linkage mapping of the RppK locus based on 192 families delimited it to the region between markers M3 and M6. The numbers below the black rectangle indicate the relative genetic distance (cM) between markers. d High-resolution linkage analysis performed by genotyping 3392 plants of a heterogeneous inbred family (HIF) delimited RppK to a 15.2 kb interval flanked by markers RRD103 and RRD111. The number of recombinants is shown below the markers. Green segments represent the K22 allele, and yellow segments represent the DAN340 allele. The names of lines and the corresponding phenotypes are provided next to the haplotype. R, resistant; S, susceptible. e The RppK region contains three predicted NLR genes, which encode CC-NB-LRR proteins. Scale bar, 1 kb. f Structure of the R3 genomic sequence construct used for generating transgenic maize plants. LB, left border; RB, right border; Bar: Bialaphos Resistance gene. The construct contains the entire R3 genomic DNA sequence, including its 3.1 kb promoter region and a 2.4 kb downstream region. The back arrow indicates the Bar gene. g , h The disease phenotypes and scores of two independent transgenic plant families carrying the R3 genomic sequence. Values are means ± SDs; n = 15, 17, 14, and 8 individual plants of positive and negative lines of family 1 and family 2, respectively. **** P < 0.0001 (Student’s t -test, two- t ailed; P = 1.2596E-15, 5.4354E-07). Source data are provided as a Source Data file. Full size image The RppK -linked molecular markers RUST7-5 and RUST9-4 were then used to screen BAC libraries of K22 and DAN340. The sequencing and annotation of five BAC clones from K22 revealed that the candidate region between markers SNP20 and SNP5 in K22 spanned 29.8 kb and contained three genes ( R1 , R2 , and R3 ) (Supplementary Fig. 3 ). The three candidate genes belong to the CC-NLR gene family with more than 96% nucleotide identity with each other (Supplementary Figs. 4 and 5 ). In contrast, the candidate region in the susceptible inbred line DAN340 was 20.2 kb and harbors only one CC - NLR gene; and, this gene was named as DAN340 R gene homologous to R3 , or DR3 (Supplementary Figs. 4 and 5 ). Based on the DNA sequences of the candidate regions in K22 and DAN340, we developed more markers to genotype recombinant plants. The candidate region for the RppK region was ultimately delimited between markers RRD103 and RRD111, which encompassed only the R2 and R3 genes (Fig. 1d, e ). We subsequently sequenced the DR3 and R3 genes in 21 recombinant plants and found that 11 of them showed recombination between DR3 and the R1 , R2 or R3 gene (Supplementary Fig. 6 ). Among the 11 recombinant lines, five lines (4H1074, 4H1505, 4H1083, 4H1028 and 4H1213) carrying the R3 gene showed resistance to SCR, whereas the other six lines, containing either no R3 gene (5H2661, 4H1285 and 4H1169) or only a partial R3 gene (4H1652, 4H1474 and 4H943), exhibited a susceptible response to SCR (Supplementary Fig. 6 ). These results indicated that R3 gene is responsible for RppK resistant against SCR. To determine whether R2 or R3 contributed to SCR resistance, we cloned genomic DNA fragments of 12.6 and 11.4 kb for R2 and R3 , respectively, from K22; these fragments contained whole genes with their native promoter and terminator sequences (Fig. 1f and Supplementary Fig. 7a ). The two fragments were then transformed into the susceptible inbred line KN5585. Two independent T 1 families of R2 or R3 gene transgenic plants were tested for resistance to natural infection by P. polysora in the field in Hainan over three years (2017, 2019 and 2020). R2 transgenic plants showed similar SCR susceptibility to the nontransgenic plants (Supplementary Fig. 7b, c ), whereas all R3 transgenic plants from two independent families showed stronger resistance to SCR than the nontransgenic plants (Fig. 1g, h and Supplementary Fig. 8 ). In order to confirm the resistance function of R3 gene, R3 transgenic plants and nontransgenic plants were inoculated with five different isolates of P. polysora in growth room (Supplementary Fig. 9a ). Moreover, R3 transgenic plants were more resistant to all five P. polysora isolates than the nontransgenic control plants (Supplementary Fig. 9b–f ). We conclude that R3 is the QTL encoding resistance gene against SCR, and was renamed as RppK . RppK presents great values for maize breeding To explore natural RppK variation in maize accessions, we used four RppK -related molecular markers (R8.65, R8.63, Del13K and R8.61) (Supplementary Fig. 10a, b ) to screen ~500 diverse maize inbred lines from an association mapping panel [48] and found that only 17 of them contained the RppK gene (Supplementary Fig. 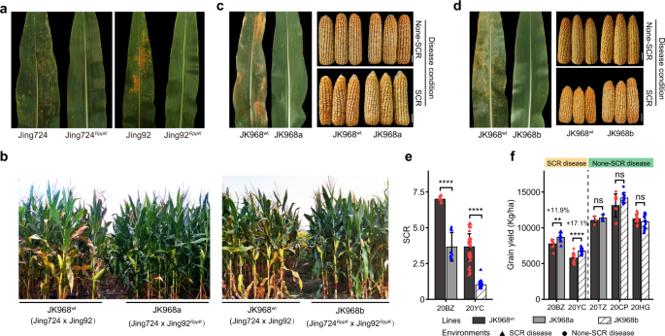Fig. 2:RppKimproves the grain yield of maize hybrid JK968 (Jing724 × Jing92) in the presence of SCR disease. aSCR disease phenotypes of wild-type lines (Jing724 and Jing92) and improved lines (Jing724RppKand Jing92RppK) carrying theRppKallele under field conditions.bThe field performance of hybrid JK968wt, improved hybrid JK968a (Jing724 × Jing92RppK) and improved hybrid JK968b (Jing724RppK× Jing92RppK) in the field in the presence of SCR disease. Hybrid JK968a was derived from a cross between Jing724 and Jing92RppKand Hybrid JK968b was derived from a cross between Jing724RppKand Jing92RppK.cSCR disease phenotypes of hybrid JK968wtand hybrid JK968a under field conditions and ear phenotypes of hybrid JK968wtand hybrids JK968a in the presence or absence of SCR disease. Scale bars = 3 cm.dSCR disease phenotypes of hybrid JK968wtand hybrid JK968b under field conditions and ear phenotypes of hybrid JK968wtand hybrids JK968b in the presence or absence of SCR disease. Scale bars = 3 cm.eThe SCR disease phenotypes of hybrids JK968wt, JK968a, and JK968b in field trials were evaluated in Bozhou (20BZ,P= 8.48818E-06) and Yongcheng (20YC,P= 1.38435E-33) China, in 2020.fThe grain yields of JK968wt, JK968a, and JK968b in the presence or absence of SCR disease in field trials in China in 2020. SCR disease conditions: 20BZ (n= 9 repeat plots; 38 plants of each line in each plot;P= 0.005498515), Bozhou, China, in 2020; 20YC (n= 16 repeat plots; 11 plants of each line in each plot;P= 1.96453E-05), Yongcheng, China, in 2020; non-SCR disease conditions: 20TZ (n= 3 repeat plots; 38 plants of each line in each plot;P= 0.4957928), Tongzhou, China, in 2020; 20CP (n= 9 repeat plots; 38 plants of each line in each plot;P= 0.100474299), Changping, China in 2020; 20HG (n= 16 repeat plots; 11 plants of each line in each plot;P= 0.212607571), Huanggang, China, in 2020. Values are means ± SDs. **P< 0.01; ****P< 0.0001 (Student’st-test, two-tailed). Source data are provided as a Source Data file. 10 , Supplementary Table 2 and Supplementary Data 1 ). Also, we screened 168 teosinte lines and 288 landrace lines using the functional marker R8.63, which did not amplify related sequences (Supplementary Data 2 and 3 ). Further, we checked 74 commercial maize hybrid lines and found that only five of them contained the RppK gene (Supplementary Fig. 11 and Supplementary Data 4 ). The low frequency of the RppK gene in the current maize collections indicates that the allele has not broadly spread in maize lines, which highlights the potential value of the RppK gene in improving SCR resistance in maize breeding. Therefore, we introgressed the RppK allele into ten elite inbred lines via backcrossing and evaluated their SCR resistance in Hainan, China. The plants harboring the RppK gene were significantly more resistant to SCR than the plants without RppK (Supplementary Fig. 12 ). To evaluate the breeding value of RppK in hybrids, we performed repeated backcrossing and molecular marker-assisted selection to introduce the RppK gene into the two parental lines of the maize hybrid JK968 (Jing724 × Jing92), which has been planted seven million hectares in China over the past decade [49] . In the field, the JK968 hybrid lines carrying RppK were more resistant to SCR than the original JK968 hybrid (Fig. 2a–d ). As a result, the grain yields of the JK968 lines carrying RppK were 11.9% (with one RppK allele, JK968a) and 17.1% (with two RppK alleles, JK968b) higher than that of the original JK968 hybrid without RppK in the presence of SCR without significant changes in major agronomic traits (Fig. 2c–f and Supplementary Fig. 13 ). We also improved the SCR resistance of four other hybrid lines with different genetic backgrounds by using the same strategy and got similar results (Supplementary Figs. 14 and 15 ). Moreover, we generated four additional hybrids by crossing transgenic KN5585 RppK lines with four maize inbred lines (B73, Mo17, IL1, and IL2). Consistent with the previous results, the RppK gene enhanced maize resistance against SCR and increased the grain yield by 4.51% to 15.6% under different SCR disease conditions with no yield penalty in the absence of SCR (Supplementary Figs. 14 – 16 ). These results indicate the high breeding value of RppK in maize. Fig. 2: RppK improves the grain yield of maize hybrid JK968 (Jing724 × Jing92) in the presence of SCR disease. a SCR disease phenotypes of wild-type lines (Jing724 and Jing92) and improved lines (Jing724 RppK and Jing92 RppK ) carrying the RppK allele under field conditions. b The field performance of hybrid JK968 wt , improved hybrid JK968a (Jing724 × Jing92 RppK ) and improved hybrid JK968b (Jing724 RppK × Jing92 RppK ) in the field in the presence of SCR disease. Hybrid JK968a was derived from a cross between Jing724 and Jing92 RppK and Hybrid JK968b was derived from a cross between Jing724 RppK and Jing92 RppK . c SCR disease phenotypes of hybrid JK968 wt and hybrid JK968a under field conditions and ear phenotypes of hybrid JK968 wt and hybrids JK968a in the presence or absence of SCR disease. Scale bars = 3 cm. d SCR disease phenotypes of hybrid JK968 wt and hybrid JK968b under field conditions and ear phenotypes of hybrid JK968 wt and hybrids JK968b in the presence or absence of SCR disease. Scale bars = 3 cm. e The SCR disease phenotypes of hybrids JK968 wt , JK968a, and JK968b in field trials were evaluated in Bozhou (20BZ, P = 8.48818E-06) and Yongcheng (20YC, P = 1.38435E-33) China, in 2020. f The grain yields of JK968 wt , JK968a, and JK968b in the presence or absence of SCR disease in field trials in China in 2020. SCR disease conditions: 20BZ ( n = 9 repeat plots; 38 plants of each line in each plot; P = 0.005498515), Bozhou, China, in 2020; 20YC ( n = 16 repeat plots; 11 plants of each line in each plot; P = 1.96453E-05), Yongcheng, China, in 2020; non-SCR disease conditions: 20TZ ( n = 3 repeat plots; 38 plants of each line in each plot; P = 0.4957928), Tongzhou, China, in 2020; 20CP ( n = 9 repeat plots; 38 plants of each line in each plot; P = 0.100474299), Changping, China in 2020; 20HG ( n = 16 repeat plots; 11 plants of each line in each plot; P = 0.212607571), Huanggang, China, in 2020. Values are means ± SDs. ** P < 0.01; **** P < 0.0001 (Student’s t -test, two-tailed). Source data are provided as a Source Data file. Full size image The RppS gene is an allele of RppK There are eight other SCR resistance QTLs mapped to the same region as RppK on the short arm of chromosome 10 [33] , [37] , [40] , [41] , [42] , [43] , [44] . We obtained resistant donor lines for five of those QTLs (CML470, CML496, P25, QI319, and SCML205) and analyzed their genetic relationships with RppK . 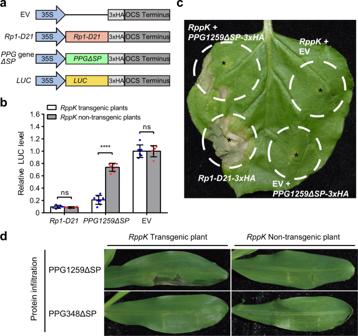Fig. 3:PPG1259is the cognate avirulence gene ofRppK. aSchematic diagrams of constructs forAvrRppKgene screening in transient protoplast expression assays. EV is the empty vector;Rp1-D21was used as the positive control;PPGgenes fromP. polysorawere cloned by using mRNA isolated fromP. polysora-infected leaves; ΔSPindicates deletion of the signal peptide region; and theLUCconstruct was used to evaluate cell viability in the transient protoplast expression assay.bPPG1259ΔSPexpression in the protoplasts ofRppKtransgenic plants induced an HR but its expression in the protoplasts of nontransgenic plants did not.PPG1259ΔSPwas coexpressed with the35s:LUCconstruct in the protoplasts ofRppKtransgenic plants or nontransgenic plants; theRp1-D21gene or empty vector (EV) was coexpressed with the35s:LUCconstruct in this assay as a positive or negative control, respectively. Relative LUC levels were measured to indicate the viability of protoplasts. Values are means ± SDs (for expression ofPPG1259ΔSP,n= 8; for the others,n= 6;P= 0.4466, 3.4E-10, 1). **P< 0.01; ns, not significant (two-tailed Student’st-test).cThe coinfiltration of the construct carrying theRppKgenomic DNA sequence with the35S:PPG1259ΔSPconstruct induced an HR inN. benthamiana. The coinfiltration of the construct carrying theRppKgenomic DNA construct or the35S:PPG1259ΔSPconstruct with the empty vector were performed as negative controls and the infiltration ofRp1-D21-3×HAwas taken as the positive control. The infiltration sites were labeled with “*”.dInfiltration of the PPG1259ΔSP protein intoRppKtransgenic plants and nontransgenic plants. GST-PPG1259ΔSP and GST-PPG348ΔSP proteins were expressed inE. coliand purified. After digestion with the 3C PPase enzyme to cleave the GST tag, PPG1259ΔSP and PPG348ΔSP were infiltrated into the leaves of 3-leaf stageRppKtransgenic plants and nontransgenic plants, respectively. In this assay,PPG348ΔSP, which did not induce a cell death phenotype in protoplasts ofRppKtransgenic plants or nontransgenic plants, was used as the negative control. Source data are provided as a Source Data file. By genotyping these lines using four markers (Del13K, R8.65, R8.63, and R8.61), we discovered that only SCML205, which carried the RppS locus, showed the same genotype as K22 (Supplementary Table 3 ). Furthermore, sequencing analysis revealed that SCML205 carried a RppK genomic DNA sequence almost identical to the RppK gene from K22, with only a 2 bp-indel difference in the second intron region between the two alleles (Supplementary Fig. 17 ). Therefore, the RppS locus from SCML205 is likely to be identical to RppK in K22. Cloning of AvrRppK from P. polysora In order to identify AvrRppK , we used PacBio sequencing to obtain the full-length mRNA sequences of P. polysora isolated from germinated urediospores. Through extensive bioinformatic analysis [50] , [51] , we identified 965 P. polysora genes ( PPGs ) predicted to encode secretory proteins, and successfully cloned 338 of them with a cysteine content greater than 1.8% (Supplementary Fig. 18 ). The recognition of an Avr protein by the corresponding R protein typically activates the hypersensitive response (HR), which is a rapid cell-death phenotype. A powerful tool for Avr gene identification has been developed based on transient protoplast expression of the LUC reporter gene, whose expression level is used as an indicator of cell viability [52] , [53] . To identify the interactor of the RppK gene, we coexpressed the 338 cloned PPGΔSPs ( PPG genes without signal peptide region) with the LUC gene in the protoplasts of transgenic RppK plants and nontransgenic control plants. Rp1-D21 , an HR-activating NLR gene [54] , was used as a positive control (Fig. 3a ). Only PPG1259ΔSP induced a strong HR in the protoplasts of transgenic RppK plants and no HR in those of nontransgenic control plants (Fig. 3b and Supplementary Fig. 19 ). Further, we deployed the transient expression system in Nicotiana benthamiana . The RppK genomic DNA clone was coexpressed with the PPG1259ΔSP gene in N. benthamiana . We observed a clear HR when the RppK and PPG1259ΔSP clones were coinfiltrated (Fig. 3c ). In contrast, no HR was triggered by the infiltration of RppK genomic DNA or PPG1259ΔSP with an empty vector (EV) (Fig. 3c and Supplementary Fig. 20 ). This indicated that RppK induced the HR in a PPG1259 -dependent manner. Moreover, we generated recombinant constructs encoding GST-PPG1259ΔSP and GST-PPG348ΔSP for the protein infiltration assay. PPG348ΔSP was used as a negative control because it did not induce cell death in maize protoplasts with or without RppK . These two constructs were expressed in Escherichia coli , and the purified recombinant proteins were digested with 3 C PPase to cleave the GST tag (Supplementary Fig. 21 ). The purified PPG1259ΔSP and PPG348ΔSP proteins were then infiltrated into the leaves of transgenic RppK plants and nontransgenic control plants. One day after infiltration, a clear HR was observed in the PPG1259ΔSP-infiltrated leaves of transgenic RppK plants but not in the PPG1259ΔSP-infiltrated leaves of nontransgenic control plants (Fig. 3d ). As expected, no HR was observed in the PPG348ΔSP-infiltrated leaves of either transgenic RppK plants or nontransgenic control plants (Fig. 3d ). So, we conclude that the interaction between PPG1259 encoded AvrRppK protein and RppK could trigger ETI. Fig. 3: PPG1259 is the cognate avirulence gene of RppK . a Schematic diagrams of constructs for AvrRppK gene screening in transient protoplast expression assays. EV is the empty vector; Rp1-D21 was used as the positive control; PPG genes from P. polysora were cloned by using mRNA isolated from P. polysora -infected leaves; Δ SP indicates deletion of the signal peptide region; and the LUC construct was used to evaluate cell viability in the transient protoplast expression assay. b PPG1259ΔSP expression in the protoplasts of RppK transgenic plants induced an HR but its expression in the protoplasts of nontransgenic plants did not. PPG1259ΔSP was coexpressed with the 35s:LUC construct in the protoplasts of RppK transgenic plants or nontransgenic plants; the Rp1-D21 gene or empty vector (EV) was coexpressed with the 35s:LUC construct in this assay as a positive or negative control, respectively. Relative LUC levels were measured to indicate the viability of protoplasts. Values are means ± SDs (for expression of PPG1259ΔSP , n = 8; for the others, n = 6; P = 0.4466, 3.4E-10, 1). ** P < 0.01; ns, not significant (two-tailed Student’s t -test). c The coinfiltration of the construct carrying the RppK genomic DNA sequence with the 35S:PPG1259ΔSP construct induced an HR in N. benthamiana . The coinfiltration of the construct carrying the RppK genomic DNA construct or the 35S:PPG1259ΔSP construct with the empty vector were performed as negative controls and the infiltration of Rp1-D21-3×HA was taken as the positive control. The infiltration sites were labeled with “*”. d Infiltration of the PPG1259ΔSP protein into RppK transgenic plants and nontransgenic plants. GST-PPG1259ΔSP and GST-PPG348ΔSP proteins were expressed in E. coli and purified. After digestion with the 3C PPase enzyme to cleave the GST tag, PPG1259ΔSP and PPG348ΔSP were infiltrated into the leaves of 3-leaf stage RppK transgenic plants and nontransgenic plants, respectively. In this assay, PPG348ΔSP , which did not induce a cell death phenotype in protoplasts of RppK transgenic plants or nontransgenic plants, was used as the negative control. Source data are provided as a Source Data file. Full size image We also coexpressed the RppS genomic DNA clone with the AvrRppKΔSP gene in N. benthamiana . A clear HR was observed when the RppS and AvrRppKΔSP clones were coinfiltrated and no HR was triggered in the controls (Supplementary Fig. 22 ). It indicates that RppS might recognize AvrRppK to trigger ETI. AvrRppK of P. polysora suppresses plant resistance AvrRppK encodes a 96-aa protein with a predicted secretion signal peptide at the N-terminus but lacks any other known structural domain. BLASTP and BLASTN analysis identified no proteins or genes with similarity to AvrRppK. Therefore, AvrRppK might only exist in P. polysora . By using single-cell sequencing technology [55] , we sequenced and annotated part of the genome of a P. polysora strain isolated from Wuhan and identified one contig (8.2 kb) containing the AvrRppK gene, which was flanked by a large number of repeat sequences (Supplementary Fig. 23 ). To evaluate the variation in AvrRppK in natural P. polysora isolates, we designed gene-specific molecular markers to examine the genotypes of more than 100 P. polysora isolates collected from corn fields in Hainan, Guangxi and Hubei provinces in China. AvrRppK gene sequences with the same size were successfully amplified from the isolates. Furthermore, we sequenced the AvrRppK coding sequences amplified from 20 isolates from Hainan, 11 isolates from Guangxi, 6 isolates from Hubei and mixed P. polysora spores from the field. Interestingly, their coding sequences of AvrRppK from all isolates were identical to the AvrRppK coding DNA sequence of the Wuhan isolate (Fig. 4a ). Therefore, the AvrRppK gene was highly conserved in P. polysora . Fig. 4: AvrRppK suppresses chitin-triggered immunity. a The AvrRppK gene is conserved in all tested P. polysora field isolates. DNA samples were isolated from twenty P. polysora isolates from Hainan, eleven isolates from Guangxi, six isolates from Hubei and mixed spores collected from Hainan, Guangxi and Hubei, respectively; b The expression level of AvrRppK during infection. Five-leaf stage B73 plants were inoculated with conidia of the P. polysora Wuhan strain. Leaf samples taken at 1, 3, 5, 7, and 9 days after inoculation (dai) were used for RT-qPCR to evaluate the expression levels of AvrRppK relative to those of the P. polysora Actin gene. Values are means ± SDs ( n = 3 repeats). One-way ANOVA with Fisher’s LSD test (mean ± SD; n = 3, biologically independent samples). Different letters indicate significant differences at P < 0.05. c The trans c ription levels of AvrRppKΔSP measured by RT-qPCR in two independent transgenic maize lines overexpressing AvrRppKΔSP ( n = 3). d The SCR disease phenotypes of two independent transgenic maize lines overexpressing AvrRppKΔSP . “+” means transgenic-positive plants, “-” means transgenic-negative plants. e The SCR disease scores of two independent transgenic maize lines overexpressing AvrRppKΔSP ( n = 7, 14, 5, 5). f The fungal biomass accumulation in two independent transgenic maize lines overexpressing AvrRppKΔSP was measured by RT-qPCR amplification of the P. polysora Actin gene relative to the Zea mays Actin gene ( n = 3). g The chitin-triggered MAP kinase activity was suppressed by AvrRppK . Western blot was used to detect MAP kinase activity by anti-Phospho-p44/42 MAPK antibody (dilution 1:1000). The loading control was maize Actin proteins measured by western blot using anti-Actin antibody (dilution 1:5000). Relative MAP kinase activity was normalized to the level of Actin protein. h Chitin-induced ROS accumulation was suppressed by AvrRppK . The absolute luminescence was used to represent ROS accumulation (for each time point, n = 6). Water treatment was taken as the control. For c – h , values are means ± SDs; * P < 0.05, *** P < 0.001, **** P < 0.0001 (two-tailed Student’s t -test). These experiments were repeated three times with the similar results. Source data are provided as a Source Data file. Full size image RT-qPCR assays showed that AvrRppK was expressed at high levels relative to the P. polysora Actin gene at 1, 3, 5, 7, and 9 days after inoculation (Fig. 4b ). To determine whether AvrRppK can enhance disease development, we generated transgenic maize plants overexpressing AvrRppK ∆ SP driven by ZmUbi promoter and RT-qPCR results confirmed the expression of AvrRppK ∆ SP in two independent lines (Fig. 4c ). After challenged with P. polysora , AvrRppK ∆ SP transgenic-positive plants in two independent lines showed more susceptible response to SCR than transgenic-negative plants (Fig. 4d, e ) and more P. polysora biomass was accumulated in AvrRppK ∆ SP transgenic-positive plants than in transgenic-negative plants (Fig. 4f ). It indicates that expression of AvrRppK can enhance the development of SCR. In order to test whether AvrRppK can suppress ETI, we coexpressed AvrRppK ∆ SP with Rp1-D21 in N. benthamiana , and clear HR was observed, similar as overexpression of Rp1-D21 alone (Supplementary Fig. 24 ), which indicates AvrRppK cannot suppress Rp1-D21 -mediated ETI. Further, we tried to test whether AvrRppK could suppress PTI. Transgenic plants overexpressing AvrRppK ∆ SP were treated with chitin and two typical PTI responses (MAP kinase signaling and ROS accumulation) were examined. As the results shown, the chitin-triggered MAP activation was suppressed in AvrRppK ∆ SP transgenic-positive plants, compared with that in transgenic-negative plants (Fig. 4g and Supplementary Fig. 25a ). Also, the chitin-triggered ROS accumulation in AvrRppK ∆ SP transgenic-positive plants was weaker than that in transgenic-negative plants (Fig. 4h and Supplementary Fig. 25b ). All of these results indicate that AvrRppK can significantly suppress chitin-triggered PTI. The ideal disease resistance in crops would be durable, broad-spectrum resistance, and with no fitness tradeoffs. Here, we reported the cloning of a maize NLR gene, RppK , for resistance against southern corn rust (SCR), and its cognate Avr gene, AvrRppK , from P. polysora (the causal pathogen of SCR). The introgression of the RppK gene into different maize inbred lines and hybrid lines significantly enhanced resistance against multiple P. polysora isolates and increased yield in the present of P. polysora . Effector proteins are major virulence factors of biotrophic and hemibiotrophic pathogens that suppress plant immunity [16] , [56] . In resistant plants, NLR proteins detect effector proteins and trigger ETI [57] . However, effector proteins are subject to rapid evolution through deletions or mutations [21] , [58] . Consequently, resistant plants may regain susceptibility to pathogens. For example, the disruption of the AvrSr35 gene by a MITE insertion in Puccinia graminis f. sp. tritici prevents recognition by the wheat NLR gene Sr35 [59] . However, the core effectors of pathogens are highly conserved and widely distributed in particular pathogens, and the mutation of a core effector significantly suppresses pathogen virulence [58] . Three core effectors in Ustilago maydis , Cce1, Pep1 and Vp1, are highly conserved in smut fungi and are required for their virulence [60] , [61] . In the present study, the coding sequences of AvrRppK were found to be identical in all tested P. polysora isolates (Fig. 4a ), and AvrRppK was highly expressed during infection (Fig. 4b ). Overexpression of AvrRppK in maize significantly suppressed maize resistance against SCR and reduced chitin-mediated PTI (Fig. 4d–h and Supplementary Fig. 25 ). All of this evidence indicated that AvrRppK might function as an effector. However, it should be noted that we didn’t provide genetic evidences to support its role as a core effector. Since core effectors are highly conserved in specific pathogens, it has been proposed that the deployment of NLR genes corresponding to core effectors is a promising strategy for achieving broad-spectrum resistance [21] . Although many core effectors have been identified by comparing the genomic DNA sequences of different strains of a specific pathogen [58] , [62] , [63] , no NLR genes recognizing these core effectors have been identified. Here, we cloned a maize NLR gene, RppK . The introgression of RppK into multiple elite maize inbred lines and hybrids significantly enhanced resistance against P. polysora and increased yields in the present of P. polysora (Fig. 2 and Supplementary Figs. 12 – 15 ). The improved maize lines were planted in different locations and were challenged with different P. polysora isolates, and the results showed that RppK functioned well in all tested locations (Supplementary Figs. 12 and 14 – 16 ). These results indicate that the deployment of a single NLR gene is sufficient to activate resistance against multiple P. polysora isolates. Although the introgression of resistance genes into crops normally causes fitness tradeoffs [64] , no yield loss in the absence of P. polysora was observed in any of the tested maize hybrid lines after the introgression of the RppK gene (Fig. 2c, d, f and Supplementary Figs. 13 – 15 ). Furthermore, several important agricultural traits were unaffected by the introgression of the RppK gene (Supplementary Figs. 13 and 14 ). All of these results confirmed that the RppK gene presents great values in maize breeding. In the 500 inbred lines, only seventeen inbred lines contains RppK gene (Supplementary Data 1 ). 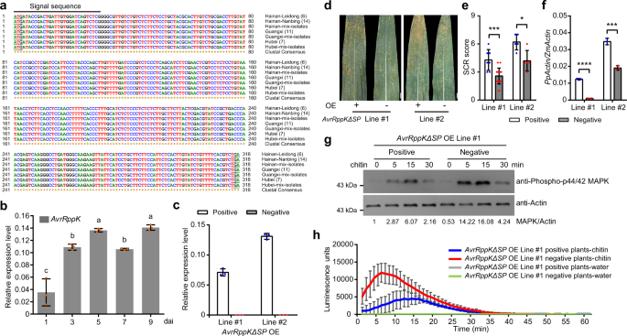Fig. 4:AvrRppKsuppresses chitin-triggered immunity. aTheAvrRppKgene is conserved in all testedP. polysorafield isolates. DNA samples were isolated from twentyP. polysoraisolates from Hainan, eleven isolates from Guangxi, six isolates from Hubei and mixed spores collected from Hainan, Guangxi and Hubei, respectively;bThe expression level ofAvrRppKduring infection. Five-leaf stage B73 plants were inoculated with conidia of theP. polysoraWuhan strain. Leaf samples taken at 1, 3, 5, 7, and 9 days after inoculation (dai) were used for RT-qPCR to evaluate the expression levels ofAvrRppKrelative to those of theP. polysora Actingene. Values are means ± SDs (n= 3 repeats). One-way ANOVA with Fisher’s LSD test (mean ± SD;n= 3, biologically independent samples). Different letters indicate significant differences atP< 0.05.cThe transcription levels ofAvrRppKΔSPmeasured by RT-qPCR in two independent transgenic maize lines overexpressingAvrRppKΔSP(n= 3).dThe SCR disease phenotypes of two independent transgenic maize lines overexpressingAvrRppKΔSP. “+” means transgenic-positive plants, “-” means transgenic-negative plants.eThe SCR disease scores of two independent transgenic maize lines overexpressingAvrRppKΔSP(n= 7, 14, 5, 5).fThe fungal biomass accumulation in two independent transgenic maize lines overexpressingAvrRppKΔSPwas measured by RT-qPCR amplification of theP. polysora Actingene relative to theZea mays Actingene (n= 3).gThe chitin-triggered MAP kinase activity was suppressed byAvrRppK. Western blot was used to detect MAP kinase activity by anti-Phospho-p44/42 MAPK antibody (dilution 1:1000). The loading control was maize Actin proteins measured by western blot using anti-Actin antibody (dilution 1:5000). Relative MAP kinase activity was normalized to the level of Actin protein.hChitin-induced ROS accumulation was suppressed byAvrRppK. The absolute luminescence was used to represent ROS accumulation (for each time point,n= 6). Water treatment was taken as the control. Forc–h, values are means ± SDs; *P< 0.05, ***P< 0.001, ****P< 0.0001 (two-tailed Student’st-test). These experiments were repeated three times with the similar results. Source data are provided as a Source Data file. Six of them belong to non-stiff stalk (NSS) group; eight of them belong to tropical-subtropical (TST) subgroup; and three of them belong to mixed subgroup (Supplementary Table 4 ) [48] . Also, eleven of the seventeen lines were originated from China, and six of them were originated from CIMMYT, Mexico (Supplementary Table 4 ) [48] . Further, only five of 74 commercial maize hybrids in China contain RppK gene (Supplementary Fig. 11 and Supplementary Data 4 ). Based on the information on https://chinaseed114.com , they were released to the market during the last 12 years. So, RppK gene is a rare allele and it has not been widely spread in maize inbred lines, which partially explain why RppK gene has been durable for more than 30 years in China. Effectors as the major virulence weapons of pathogens and NLR proteins as the major components of the plant immune system are subjected to evolutionary pressure [65] , which consequently results in high variation in effectors and NLR proteins [16] , [21] . Core effectors are widely distributed in a particular pathogen [21] , [58] . It indicates that pathogens cannot afford to lose them [58] . To evade the recognition by host resistance proteins, some core effectors show polymorphism in different isolates. Multiple Avramr1 homologs were identified from different P. infestans isolate and they are recognized by different Rpi-amr1 alleles [66] . In order to explain why core effectors are not deleted in the arm-race, more studies on NLR proteins and core effectors should be conducted in future. Plant materials The resistant inbred line K22, derived from K11 × Ye478 cross, is an elite subtropical line and has been used for breeding program in China for ~30 years [67] . The susceptible donor DAN340, with good agronomic traits, is one of the main inbred lines from the Luda Red Cob group in China. The F 6:7 RIL population of 192 lines was generated by crossing K22 with DAN340, followed by subsequent self-pollination [45] , [46] . The K22 × DAN340 (KD) RILs and their parental lines were planted at Sanya (109.2 °N, 18.3 °E), Hainan Province, China in 2011, 2012, and 2013 and at Xinxiang (113.9 °N, 35.3 °E), Henan Province, China in 2014. Two repeats were planted at each location in 2011, 2013 and 2014, and one repeat was planted in 2012. KD RILs and their parental lines were planted in a randomized complete block design. The association mapping panel (AMP) containing 500 diverse maize inbred lines has been reported previously [48] . The AMP lines were planted from 2011 to 2016 at three locations with a randomized complete block design. The panel lines were planted with one repeat in 2011, 2012, 2015, and 2016 and three repeats in 2013 at Sanya in Hainan Province. The lines from the same panel were planted with two repeats in two trials (i.e., Nanning (108.4 °N, 22.8 °E) in China in 2011, 2012, and Xinxiang in 2014). All lines were grown in 3.0 m row spaced 0.67 m apart with a planting density of 45,000 plants ha −1 . Disease scoring in the field The conditions with warm temperature and high humidity in Hainan Province were favorable for SCR development. The mapping lines of RIL populations were naturally infected along with DAN340 and BY815 as the susceptible control and K22 as the resistance control. The SCR phenotype was scored at the third or fourth weeks after pollination. Using the following one-nine-point scale: “1”, no disease symptom or only hypersensitivity response; “2”, 5–10% leaf area infected; “3”, 15–20% leaf area infected; “4”, 30–40% leaf area infected; “5”, 50% leaf area infected; “6”, 60% leaf area infected; “7”, 70% leaf area infected; “8”, 80–90% leaf area infected; and “9”, the whole leaf infected and dead (Supplementary Fig. 1b ). The best linear unbiased predictor (BLUP) values for each RIL and AMP lines were calculated according to the methods with minor modification [46] . The BLUP values of KD RIL were used for QTL mapping by composite interval method [68] . Inoculation in greenhouse Maize plants were planted in the Greenhouse at Huazhong Agricultural University. The inoculation with P. polysora urediospores was followed by the leaf method with minor modifications [69] . Urediospores of P. polysoda were collected from susceptible lines in Nanbing Farm, Hainan Province. The spores were brushed down from susceptible leaves with brush pens into 20 ml distilled water with one drop of Tween-20. The spores were completely suspended and adjusted to a final concentration of 5 × 10 5 spores/ml. The fully extended leaves of B73, transgenic-positive and negative plants at the 6-leaf stage were painted with spore suspension. The temperature in the greenhouse was set from 25 to 30 °C. All lines were covered with non-permeable plastic films on the top to keep high humidity. The disease symptom with pinpoint spots was observable at one week after inoculation. The experiment was repeated at least three times with similar results. BAC library screening and sequence analysis The BAC library of resistant line K22 was constructed at The Genome Resource Laboratory at Huazhong Agricultural University. Etiolated seedlings, grown in the dark for 2–3 weeks, were collected and frozen in liquid nitrogen. The BAC library was constructed using the standard protocols [70] . A total of 120960 clones were obtained and were saved individually in 315 384-well-plates with an average insertion size of 150 kb. Five positive BAC clones carrying RppK gene were identified by using PCR primers, RUST7-5 and RUST9-4 and were further confirmed with PCR amplification by primers, RRD39, RRD44, RUST8-2, RRD15, and RRD64, followed by sequencing of the PCR fragments. DNA of the five positive BAC clones were extracted using Large-Construct Kit (QIAGEN, Cat No. 12462) and was used for construction of a 20 kb insertion library for PacBio RSII. SMRT sequencing was performed in one SMRT Cell on a PacBio RSII instrument. After filtering the adaptor and low-quality reads in the raw sequencing reads, the clean data were assembled using SMRT analysis software. The contiguous sequence of about 230 kb for the genomic fragment was obtained from those BAC clones. The sequence of the target region containing three NLR genes, R1 , R2 and R3 , were confirmed again by Sanger sequencing. The BAC library screening and BAC clone sequencing of inbred line 1145 was performed similarly to that of K22. Two positive BAC clones covering the candidate region were identified and sequenced. The sequence results showed that the candidate region in line 1145 is 117 kb. The BAC library of maize inbred line DAN340 was constructed from young ear tissue [70] . To optimize cost and efficiency without sacrificing time and coverage, we combined BAC clones to make superpools and after the genomic DNA fragment by partial digestion inserted them into pIndigoBAC536-S vector. Those superpools were constructed in two dimensions for each plate in multiple copied and positive clones were identified using primers: RUST7-5 and RUST9-4. The positive superpools were diluted and spread onto culture for screening of positive clones using the same primers. One positive BAC clone was identified by utilization of this strategy and was amplified by polymorphism markers to deduce the covered length. This single BAC clone from inbred line DAN340 was sequenced by Pacific Biosciences single-molecule sequencing as described above and was found to contain a 102 kb genomic fragment insertion. The repetitive elements in the genomic sequences of candidate region were analyzed by using RepeatMasker Web Server ( www.repeatmasker.org/ ). Gene annotation were analyzed by using the coding sequences of the B73 reference genome (AGPv2, FGS 5b [71] ) with GMAP package (version 2015-09-29 [72] ). The gene finding programs including GENSCAN and Fgenesh were also used [73] , [74] . Those results were combined together manually. The sequence comparison between homology regions of RppK locus was done by using BLASTN suite from the National Center for Biotechnology Information. The graphical display of alignment was drawn with genoPlotR package (version 0.8.2) [75] . Breakpoint detection in recombinant families To confirm the breakpoints in recombinant lines between RRD103 and RRD111, they were first genotyped with primers R8.63 and R8.61 to confirm the allele on the R3 promoter and then tested for the presence of the R1 and R2 genes using primer R8.65. The results were verified by sequencing PCR products as follows: presence of both R1 and R2 genes, double peaks at the nucleotides 662, 676 and 694 (relative to ATG of R2 gene) in sequencing chromatogram; presence of only R1 gene, single peaks at those sites and “ACA” haplotype; presence of only R2 gene, single peaks at those sites but “TGG” haplotype (Supplementary Fig. 10b, c ). Based on the result of R8.63, R8.61 and R8.65, the recombination model of families was constructed. Furthermore, the R8.53 PCR products of recombination families were sequenced and were aligned with R1 , R2 , R3 , and DR3 of BAC sequences. For those families in which no breakpoint in R8.53 region was identified, they were sequenced again with R8.65F/R8.64F or R8.63R/R8.64F based on the model. Those families in which the breakpoint occurred in the last intron of NLR genes, they were not used for future analysis. Transgenic maize generation and functional validation R2 and R3 genomic fragments from BAC clones were subcloned into vector pZZ01523 and the positive clones were confirmed by sequencing. The transgenic construct (pMA138) contained the genomic sequence of R3 gene (11443 bp) including 3086 bp promoter and 2378 bp downstream regions (Fig. 1f ). The transgenic construct (pMA115) contained the genomic sequence of R2 gene (12611 bp) including 4703 bp promoter and 4464 bp downstream region (Supplementary Fig. 7a ). Both pMA138 and pMA115 were transferred into KN5585, a SCR susceptible maize inbred lines, by the gene transformation platform of China National Seed Group. All the positive genomic transformation plants were self-crossed or backcrossed to KN5585. Transgenic plants were grown in Transgenic Experimental Farm of Beijing Academy of Agriculture and Forestry at Sanya, Hainan Province. Those plants including transgenic-positive plants and transgenic-negative plants were identified in each generation with R2 - and R3 -specific primers and were infected under natural inoculation. The procedures for SCR testing including the investigation time and standard of disease scores were the same as those used for RILs. The progeny-test assay was done in different genetic background populations. Statistically significant difference between transgenic and nontransgenic subgroups was determined by Student’s t -test with P -value < 0.05. PPG1259 CDS region without the signal peptide ( PPG1259 ∆ SP ) driven by ZmUbiquitin promoter was cloned into pZZ01523. The positive clone was confirmed by sequencing and was transferred into KN5585 by the gene transformation platform of Weimi Biotechnology Co., Ltd. Cell-death assay in maize protoplasts Maize protoplasts were isolated from 10 days old plants for transformation using PEG-calcium transfection of plasmid DNA and protoplast culture [76] . Constructs expressing candidate genes were co-transfected with the plasmid containing firefly Luciferase ( Luc ) gene into maize protoplasts as described before [77] . The concentrations of each plasmid and each protoplast sample were kept at the same level for all repeats and experiments. For each construct, three technical repeats were used. At 24 h after transformation, the protoplast viability was checked under fluorescence microscope (Leica). Luciferase activity was measured and quantified using a luciferase assay system (Promega). All of those experiment was repeated three times. Data were analyzed by GraphPad Prism 8 software. The experiment was repeated at least three times with similar results. RT-qPCR assay Maize inbred line B73 at five-leaf stage was inoculated with P. polysora urediospores under high-humidity conditions. mRNA was isolated from leaf samples collected at different time points after inoculation by using Trizol (Invitrogen). Moreover, RT-qPCR was done by using SYBR premix (TaKaRa) on real-time PCR (CFX96 Real-Time System, Bio-Rad). All of the experiments were done at least three times. Primers for detecting the expression levels of AvrRppK are listed in Supplementary Data 5 . For each assay, the experiment was repeated at least three times with similar results. Single-cell DNA whole-genome sequence of P. polysora For the single-cell DNA whole-genome sequencing, more than one hundred urediospores from a single uredium of P. polysora were picked up by needles under microscope. DNA from those spores were isolated by using the QIAGEN REPLI-g Single-Cell Kit and DNA amplification was done by MDA following the standard protocol [55] . The whole-genome amplification products were submitted for detection and sequencing. Identification of effector candidate genes in P. polysora P. polysora urediospores collected from inoculated leaves in greenhouse were evenly dispersed on the surface of sterile water and kept at room temperature for 24 h. Then the mycelia were collected and washed three time by sterile water. RNA was isolated from the collected mycelia by Trizol (Invitrogen) and was submitted for Pacbio sequencing (Shanghai Personal Biotechnology Co., Ltd). The sequence results were analyzed by SMRT analysis (V2.3) and 53296 full-length sequences were identified [50] . The full-length transcripts were transcribed by Transdecoder v4.1.0 and signal peptide in ORF were analyzed by SignaIP-4.0 [51] . The analysis identified 965 secretory proteins and 338 of them were successfully cloned. Transient expression in N. benthamiana For transient expression assay in N. benthamiana , constructs were transformed by electroporation into the Agrobacterium strain GV3101 and positive Agrobacterium transformants were identified by PCR using primers specific to each construct. Agrobacteria were inoculated into LB medium and grown overnight at 28 °C with shaking. Agrobacterium cultures were collected by centrifugation at 4602 × g for 10 min and the bacterial pellet were resuspended in the infiltration buffer (10 mM MES, 10 mM MgCl 2 and 200 µM acetosyringone) and adjusted to OD 600 of 0.5 before infiltration into the leaves of 30-day old N. benthamiana . Leaves of N. benthamiana for transient expression. HA tagged proteins were detected by western blot using anti-HA antibody (Abcom, Cat#49969, dilution 1:1000). The experiment was repeated at least three times with similar results. Expression and purification of recombinant proteins in E. coli For expression and purification of GST recombinant proteins in E. coli , the coding DNA sequences of PPG1259 and PPG348 without the signal peptide were cloned into the GST expression vector pGEX-4T-1. The recombinant constructs were transformed into home-made E. coli BL21 competent cells. The expression of recombinant proteins in E. coli was induced by adding isopropyl-b-D thiogalactopyranoside (IPTG) and the purification of proteins was performed according to the manufacturer’s manual. The purified proteins were digested by 3C PPase to cleave the GST tag. For the protein infiltration assay, two-week old seedlings of RppK -positive transgenic and negative transgenic plants from the same transgenic line were used. Purified PPG1259ΔSP and PPG348ΔSP proteins were diluted to 0.2 mg/ml in 1× PBS buffer and infiltrated into the first leaf of RppK -positive and negative transgenic plants using 1 ml syringe. The hypersensitive response (HR) was evaluated at 24 h after infiltration. The experiment was repeated at least three times with similar results. ROS detection assay and MAPK kinase activity assay For ROS detection assay, two independent PPG1259ΔSP transgenic lines at three-leaf stage were tested in this assay. Leaf discs were taken by using a 4 mm diameter punch. All discs were put in 1% DMSO for overnight, then 1% DMSO was replaced by 2× L-012 in 0.005% Silwet L-77 and disc samples were treated for 1 h. Two kinds of 2× HRP buffer were prepared; one was for the treatment buffer containing 50 mg/ml chitin and the other was for the mock control without chitin. Next, eight cells were treated with treatment buffer and the others were treated with the mock buffer. A microplate detector was used to collect light signals, which reflected ROS production. The signal was read every one minute for one hour and the data were analyzed to display the changes of ROS production over time. The experiment was repeated at least three times with similar results. Moreover, statistical tests were done by two-tailed Student’s test with P < 0.05. For chitin-induced MAPK kinase activity assay, two independent PPG1259ΔSP transgenic lines at six-leaf stage were tested in this assay. The fully extended leaves were treated with 50 mg/ml chitin for 0, 5, 15, or 30 min. Then leaf samples were grounded for protein extraction. Equal amount of proteins was loaded onto a 12% SDS-PAGE gel for western blot. MAPK kinase activity was examined by using anti-phospho-p44/42 antibody (Cell Signaling Technology, 9101S, dilution 1: 1000) and the loading actin control was examined by using anti-Actin antibody (ABclonal, AC009, dilution 1: 5,000). Relative MAP kinase activity was normalized to the level of Actin protein. The experiment was repeated at least three times with similar results. Statistical tests were done by two-tailed Student’s t -test with P value < 0.05. Molecular breeding of RppK The cultivar K22 carrying RppK was crossed with two parental inbred lines of JK968 (Jing724 × Jing92), an elite hybrid widely planted in China, and backcrossed four time with recurrent parents to generate the BC 4 F 1 plants, which self-crossed two time to generate the BC 4 F 3 lines. Molecular markers were used to maintain the K22-derived RppK locus. Two pairs of near isogenic lines (NILs): Jing724 RppK and Jing724, Jing92 RppK and Jing92 were selected from the BC 4 F 3 progenies. Selected Jing724 RppK and Jing92 RppK carrying the RppK locus were genotyped with Genotyping-by-Sequencing and found to contain 97.4% and 96.9% of their respective recurrent parent genome. The Jing724 RppK and Jing92 RppK lines were crossed to generate the improved hybrid JK968a (Jing724 × Jing92 RppK ) and JK968b (Jing724 RppK × Jing92 RppK ). The improved IL4 RppK line was selected with similar molecular assisted selection. The inbred line IL3 was crossed with IL4 or improved IL4 RppK to generate the original Hybrid2 wt or the improved Hybrid2 RppK (IL3 × IL4 RppK ). The inbred lines: Jing72464, JingMC01 and Jing88 were respectively crossed with inbred line Jing2416 and Jing2416K (with the same RppK locus as K22), respectively, to generate paired hybrids: MC121 wt and MC121 RppK , JNK728 wt and JNK728 RppK , JNK828 wt and JNK828 RppK . To test the performance of hybrids in the field, we planted those hybrids in fields for yield tests under two conditions: a) none-SCR condition: fields in Tongzhou (116.6 °N, 39.9 °E), Changping (116.2 °N, 40.2 °E) and Huanggang (114.9 °N, 30.5 °E), China, in 2020; b) SCR condition: natural SCR nursery fields in Bozhou (115.8 °N, 33.9 °E) and Yongcheng (116.4 °N, 33.9 °E), China in 2020. Field trials of hybrids JK968 and JK968a were conducted in three locations: Bozhou, Tongzhou and Changping. Field trials for hybrids MC121 wt and MC121 RppK , JNK728 wt and JNK RppK , JNK828 wt and JNK828 RppK were done in two locations: Bozhou and Tongzhou. Each line was planted in nine subplots and each subplot contains two rows. Each row was 5 m long and spaced 60 cm with 19 plants. Field trials of hybrids JK968 and JK968b, Hybrid2 wt and Hybrid2 RppK were conducted in two locations: Yongcheng and Huanggang. Each line was planted in sixteen subplots and each subplot contains one row. Each row was 3 m long and spaced 50 cm with 11 plants. The agronomic traits (flowering time, plant height and ear height) of each line were investigated. All ears were harvested and dried to uniform moisture for scoring ear and grain traits. Yield-related traits (ear length, ear diameter, ear weight and kernel weight per plant) in a subplot were calculated. Statistically significant difference between wild-type lines and improved lines was evaluated by two-tailed Student’s t -test with P -value < 0.05. The transgenic-positive line KN5585 RppK and negative line KN5585 Wt were crossed with four inbred lines (B73, Mo17, IL1, and IL2) to generate F 1 hybrids. Those hybrids were planted in Sanya, China in 2019 to test the yield performance. Each hybrid line was planted eight rows and each row was set as one subplot. The SCR score and yield-relative traits were investigated. Statistically significant difference between hybrid line without RppK gene and improved hybrid lines with RppK gene was evaluated by two-tailed Student’s t -test with P value < 0.05. Reporting summary Further information on research design is available in the Nature Research Reporting Summary linked to this article.